Titanium dioxide nanomaterials cause endothelial cell leakiness by disrupting the homophilic interaction of VE–cadherin The use of nanomaterials has raised safety concerns, as their small size facilitates accumulation in and interaction with biological tissues. Here we show that exposure of endothelial cells to TiO 2 nanomaterials causes endothelial cell leakiness. This effect is caused by the physical interaction between TiO 2 nanomaterials and endothelial cells’ adherens junction protein VE-cadherin. As a result, VE-cadherin is phosphorylated at intracellular residues (Y658 and Y731), and the interaction between VE-cadherin and p120 as well as β-catenin is lost. The resulting signalling cascade promotes actin remodelling, as well as internalization and degradation of VE-cadherin. We show that injections of TiO 2 nanomaterials cause leakiness of subcutaneous blood vessels in mice and, in a melanoma-lung metastasis mouse model, increase the number of pulmonary metastases. Our findings uncover a novel non-receptor-mediated mechanism by which nanomaterials trigger intracellular signalling cascades via specific interaction with VE-cadherin, resulting in nanomaterial-induced endothelial cell leakiness. The pervasive use of nanomaterials (NM) generated public concerns about their possible health effects and has prompted much scientific investigation [1] . The new science of nanobiology requires greater understanding in the interaction of nanoscale particles with biological components. Due to their nano dimensions, it is possible that some of these NM enter into the circulatory system and accumulate in major organs [2] . Endothelial cells line blood vessels in many highly vascularized organs and function as gatekeepers for nutrients, waste and cell movement. The subtle control of blood vessel integrity is so important that its dysfunction is implicated in tumour angiogenesis and metastatic migration [3] , [4] . Much of this control occurs right at the adherens junctions between endothelial cells. These adherens junctions do not merely juxtapose neighbouring cells but act as intracellular signalling conduits determining cell position, proliferation, apoptosis and vascular homeostasis [5] . When this junctional continuity is disrupted, the space between adjacent endothelial cells increases to at least 1–2 μm, resulting in endothelial cell leakiness (ECL) or in an in vivo setting, vascular leakiness [3] . Species like vascular endothelial growth factor (VEGF), thrombin, angiopoietin-like 4 protein [4] and histamine [5] can perturb this tightly regulated intercellular and intracellular homeostasis and result in ECL. Toxic metal oxide NM are known to be endocytosed and induced oxidative stress [6] , [7] ; indirectly leading to ECL [8] . However, we postulate a novel mechanism where ECL can occur without uptake of NM but by virtue of their small dimensions, NM can migrate into and disrupt the adherens junction between endothelial cells. This postulated mechanism would also suggest a novel non-receptor-binding mechanism that directly causes ECL. TiO 2 –NM induce ECL We observed that a relatively benign and commonly found TiO 2 –NM actually caused ECL of an otherwise confluent layer of endothelial cells. We tested commercially available spherical-shaped TiO 2 –NM with primary particle size of 23.5 nm ( Supplementary Fig. S1 ). Hydrodynamic size measurement of TiO 2 –NM showed that these NM formed small aggregates with an average size of 57.1 nm in complex cell culture medium ( Supplementary Fig. S1 ). NM disaggregate and shed off materials when in complex aqueous environments [9] . This etches the aggregates down to smaller sizes [10] . Though generally considered to be of low cytotoxic risk [6] , we observed that TiO 2 –NM with concentration as low as 10 μM induced ECL (red arrowheads) within a short 30 min of exposure ( Fig. 1a ). This NM-induced ECL effect was sustained after 60 min of treatment ( Fig. 1a ). On the contrary, micro-sized TiO 2 (680 nm) at the same dosage range and exposure duration did not cause any observable disruption of endothelial cell layer ( Supplementary Fig. S2 ), thus supporting the notion that the observable ECL is highly dependent on primary particle size. To quantify leakiness, we plated a confluent layer of endothelial cells over 0.4 μm pores Transwell inserts and treated the cells with either TiO 2 –NM (23.5 nm) at various concentrations, TiO 2 microparticles (680 nm) and 2.5 mM EDTA (as positive control for endothelial cells leakiness). We again observed significant levels of leakiness when treating the cells with TiO 2 –NM as low as 10 μM concentrations ( Fig. 1b ) but not in the TiO 2 microparticles group ( Fig. 1b ). This size effect difference is also reported by comparative cytotoxicity studies between fine and ultrafine materials [11] but not as the cause of ECL. We tested two other similarly sized NM, silicon dioxide and silver, and observed that these two other NM also caused ECL ( Fig. 1c ). As ECL occurs at the adherens junction, one would logically deduce that the entities holding the adherens junction might be critically affected either directly or indirectly by TiO 2 –NM. Each neighbouring endothelial cell contributes one arm of VE–cadherin dimer to form a homophilic trans -interacted VE–cadherin complex. A series of these VE–cadherin complexes aligns itself to form a pericellular zipper-like structure along an intact inter-endothelial cell junction border [5] . Where ECL has occurred coincided with the loss of this zipper-like structure ( Fig. 1a ). The observation that TiO 2 –NM caused microscopic ECL further reinforced the notion that the homophilic interacted pairs of VE-cadherin were disrupted. This size factor of NM provided some clue to the mechanism. Uncovering the mechanism of how NM induce ECL would have significant biological significance as ECL is involved in cancer metastasis and progression [3] , edema and diabetic retinopathy [12] . 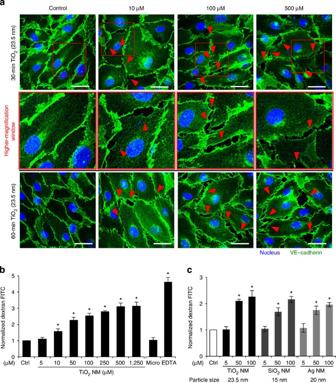Figure 1: TiO2–NM induce ECLin vitro. (a) TiO2–NM induced ECL within 30 min of exposure and this effect persisted for at least 60 min of exposure. ECL (red arrowhead) was observed on a confluent monolayer endothelial cells treated with various concentrations of TiO2–NM. Higher magnification windows showed leakiness between cells. Adherens junctions VE–cadherin visualized with immunofluorescence (green) and nuclei by 4',6-diamidino-2-phenylindole (blue). Scale bar, 50 μm. (b,c) ECL semiquantitative transwell assay showed increased leakiness after treating with TiO2–NM (23.5 nm), SiO2–NM (15 nm) and Ag–NM (20 nm). Data are means±s.d.,n=3. Student’st-test, *P<0.05. Figure 1: TiO 2 –NM induce ECL in vitro . ( a ) TiO 2 –NM induced ECL within 30 min of exposure and this effect persisted for at least 60 min of exposure. ECL (red arrowhead) was observed on a confluent monolayer endothelial cells treated with various concentrations of TiO 2 –NM. Higher magnification windows showed leakiness between cells. Adherens junctions VE–cadherin visualized with immunofluorescence (green) and nuclei by 4',6-diamidino-2-phenylindole (blue). Scale bar, 50 μm. ( b , c ) ECL semiquantitative transwell assay showed increased leakiness after treating with TiO 2 –NM (23.5 nm), SiO 2 –NM (15 nm) and Ag–NM (20 nm). Data are means±s.d., n =3. Student’s t -test, * P <0.05. Full size image Induced ECL is independent of oxidative stress or apoptosis The canonical perpetrator of NM-induced toxicity is oxidative stress [6] . Metal oxide NM, like ZnO and CuO, can induce elevation of intracellular reactive oxygen species (ROS) [6] , which indirectly cause ECL through cytoskeletal damage [8] or indirectly by activating apoptotic events, resulting in cellular shrinkage. Therefore, initially we checked whether TiO 2 –NM-induced ROS generation may have caused ECL. However, we observed significant elevation of ROS only after a time period ( Fig. 2a ) that far exceeds our initial observation of ECL at a very brief TiO 2 –NM treatment time of 30 min ( Fig. 1a ). 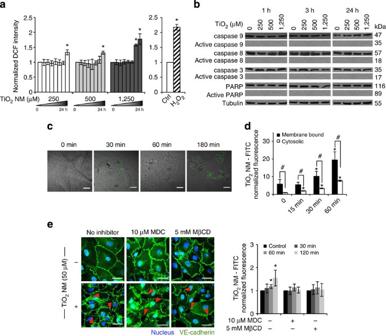Figure 2: TiO2–NM-induced ECL is independent of ROS formation, apoptosis and endocytosis (a) Significant levels of ROS upregulation in the TiO2–NM-treated cells were detected far later than the 30 min when leakiness was observed. H2O2(200 μM, 2 h) served as positive control. Graded shaded triangles represent increasing time points of 0, 0.5, 1, 2, 4, 8, 12 and 24 h. Data are means±s.d.n=3. Student’st-test compared with untreated control, *P<0.05. (b) Immunoblotting analysis of apoptosis markers showed no evidence of apoptosis over various concentrations of TiO2–NM and time points. (c) FITC-conjugated TiO2–NM (1,250 μM) were used to visualize the uptake of TiO2–NM into endothelial cells. Merged phase contrast and confocal images showed there was significant uptake (180 min) only much later than the time of ECL (30 min,Fig. 1a). Scale bar, 25 μm. (d) Cells were treated with 250 μM TiO2–FITC and the membrane and cytosolic fractions’ TiO2–FITC content measured. Normalized to cytosolic fraction att=0. There were consistently increasing amounts of TiO2–FITC associated with the membrane fraction up to 60 min. Data are means±s.d.n=3. Student’st-test, compared with corresponding cytosolic sample#P<0.05; compared tot=0 group, *P<0.05. (e) Blocking endocytosis with inhibitors did not prevent leakiness. Red arrowheads indicate the presence of ECL on endothelial cells monolayer. Scale bar, 50 μm. Data are means±s.d. ofn=3. Student’st-test, compared with no-inhibitor control, *P<0.05. Figure 2: TiO 2 –NM-induced ECL is independent of ROS formation, apoptosis and endocytosis ( a ) Significant levels of ROS upregulation in the TiO 2 –NM-treated cells were detected far later than the 30 min when leakiness was observed. H 2 O 2 (200 μM, 2 h) served as positive control. Graded shaded triangles represent increasing time points of 0, 0.5, 1, 2, 4, 8, 12 and 24 h. Data are means±s.d. n =3. Student’s t -test compared with untreated control, * P <0.05. ( b ) Immunoblotting analysis of apoptosis markers showed no evidence of apoptosis over various concentrations of TiO 2 –NM and time points. ( c ) FITC-conjugated TiO 2 –NM (1,250 μM) were used to visualize the uptake of TiO 2 –NM into endothelial cells. Merged phase contrast and confocal images showed there was significant uptake (180 min) only much later than the time of ECL (30 min, Fig. 1a ). Scale bar, 25 μm. ( d ) Cells were treated with 250 μM TiO 2 –FITC and the membrane and cytosolic fractions’ TiO 2 –FITC content measured. Normalized to cytosolic fraction at t =0. There were consistently increasing amounts of TiO 2 –FITC associated with the membrane fraction up to 60 min. Data are means±s.d. n =3. Student’s t -test, compared with corresponding cytosolic sample # P <0.05; compared to t =0 group, * P <0.05. ( e ) Blocking endocytosis with inhibitors did not prevent leakiness. Red arrowheads indicate the presence of ECL on endothelial cells monolayer. Scale bar, 50 μm. Data are means±s.d. of n =3. Student’s t -test, compared with no-inhibitor control, * P <0.05. Full size image A hallmark manifestation of apoptosis is cellular shrinkage from neighbouring cells [13] . Early report showed that TiO 2 –NM could trigger the apoptotic pathway in another cell type, mouse epidermal JB6 cells, after 180 min of TiO 2 –NM treatment [14] ; which is far later than our initial detection of ECL at 30 min. So we again checked whether apoptosis triggered by TiO 2 –NM caused ECL. Based on non-cleavage of important caspases ( Fig. 2b ), like caspases 3, 8 and 9, and also poly (ADP-ribose) polymerase, we concluded that apoptosis cannot be a cause for this type of ECL. As intracellular processes, such as ROS generation and apoptosis, cannot explain the observed ECL, we postulate that the trigger might be pre-endocytotic or extracellular. Using TiO 2 –NM covalently tagged with fluorescein isothiocyanate (FITC) and monitoring its time-dependent endocytosis, we observed significant uptake of TiO 2 –NM 180 min after exposure ( Fig. 2c ), noticeably far later than our ECL observation at 30 min post NM treatment ( Fig. 1a–c ). Next, we quantified the cellular uptake of TiO 2 -FITC in membrane and cytosolic fractions, and showed that TiO 2 –NM was mostly in the membrane fraction within the time scale of ECL ( Fig. 2d ). In order to further show that uptake is not necessary for the occurrence of the ECL, we blocked endocytosis with 10 μM monodansylcadaverine (MDC) or 5 mM methyl-β-cyclodextrin (MβCD), and that did not prevent ECL induced by 50 μM TiO 2 –NM ( Fig. 2e ). The same phenomenon was observed when cells were treated at a higher concentration of 250 μM TiO 2 –NM instead ( Supplementary Fig. S3 ). Control experiments for endocytosis inhibition ( Fig. 2e ) showed that endocytosis was indeed inhibited and at 30 min there was also insignificant uptake of TiO 2 -FITC ( Fig. 2e ). Collectively, our data strongly suggest that the cause of this ECL must have occurred before any significant TiO 2 –NM endocytosis and that the observed ECL is of extracellular and membraneous origin. TiO 2 –NM directly bind VE–cadherin in adherens junctions We observed that early ECL is not dependent on endocytosis ( Fig. 2c–e ) and TiO 2 –NM treatment profoundly resulted in leakiness while TiO 2 microparticles did not ( Fig. 1a ). Considering the known biology of adherens junctions, we reasoned from our experimental evidences and hypothesized that TiO 2 –NM by virtue of its size may have migrated into the nano-range size of the adherens junction (determined minimally by the length of a homophilically interacted complex of cadherin of ~22.5 nm. [15] It then directly binds to and disrupt the extracellular homophilic interaction of VE–cadherin, the key molecule that maintains endothelial cell–cell integrity. We tested our direct binding hypothesis and the necessity of an intact adherens junction ( a priori condition for any intact cell-cell contact) by modifying a standard protein pull-down assay but using TiO 2 –NM as a precipitation agent ( Fig. 3a ). To determine whether intact adherens junctions are necessary and to control for the artefactual situation where binding of VE–cadherin with TiO 2 –NM has instead occurred in lysis condition, we included a group where protein extracts were only exposed to TiO 2 –NM after cells were lysed (P, post-lysis group). VE–cadherin was indeed pulled down by TiO 2 –NM in a dose-dependent fashion, while the other controls (no-beads control (C) and agarose mock pulled-down control (A), post-lysis control (P) and TiO 2 microparticles-treated group) did not ( Fig. 3a ). Tight junction protein claudin-5, found in inter-endothelial niche, however, was not pulled down by TiO 2 –NM ( Fig. 3a ). Intracellular proteins, like SOD1 and tubulin, were not pulled down as well ( Fig. 3a ). This suggests some specificity of TiO 2 –NM towards VE–cadherin and again suggests involvement of the adherens junction. The observations that the post-lysis TiO 2 treatment group (P) and microparticle-treated group did not pull down any detectable VE-cadherin suggest that the in situ juxtaposition of VE–cadherin within an intact adherens junction is required for this binding and it is not merely direct physical interaction between VE–cadherin and TiO 2 –NM in a post-lysis scenario. We further showed that there is a physical interaction in situ between VE–cadherin and TiO 2 –NM by modifying a relatively new molecular interaction technique called proximity ligation assay (PLA), used mainly to prove direct protein–protein interaction ( Supplementary Fig. S4 ). We showed with modified PLA protocol that IgG-conjugated TiO 2 –NM interacted with VE–cadherin (<40 nm apart) physically ( Fig. 3b ). Implicitly observed in the images ( Fig. 3b ) is that this interaction is along the adherens junction region and occurred in situ and not in the lysed state. To further prove the distance sensitivity of the PLA technique, the negative control pair, VE–cadherin and actin which are close by but separated by α-catenin [5] complexes were utilized, and as predicted no positive PLA signals was observed ( Fig. 3b ). 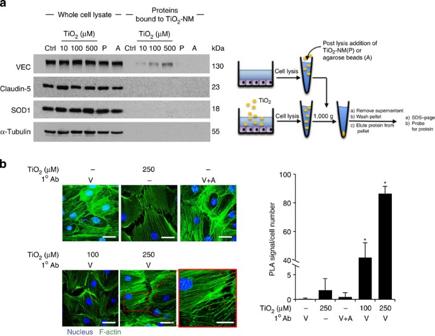Figure 3: TiO2–NM directly bind to adherens junctional homophilic VE–cadherin. (a) The presence of TiO2–NM pulled down VE–cadherin (VEC) in a dose-dependent manner. Post lysis (P), addition of TiO2–NM (1,250 μM) to a non-treated control did not pull down any detectable VE–cadherin. This suggested that an intact adherens junction is important for TiO2–NM to bind to VE–cadherin. This showed that TiO2–NM binds to VE–cadherin within the adherens junction and not in the lysis buffer condition. Protein A Agarose beads (A) were added to show that no detectable VE–cadherin were precipitated without addition of TiO2–NM. Whole cell lysate showed similar expression of VE–cadherin across the various groups, which indicated that TiO2–NM did not affect cellular VE–cadherin expression transcriptionally or post-translationally. Schematic cartoon showing the experimental setup. (b) Direct interaction between TiO2–NM and VE–cadherin was assessed with modified PLA (Supplementary Fig. S4). Intact monolayer of endothelial cells was treated with mouse-IgG-conjugated TiO2–NM for 30 min. Through the PLA protocol, red fluorescence signals were observed following mouse IgG-conjugated TiO2–NM treatments (100 and 250 μM), thus showing direct interaction. Untreated control, NM nonspecific control and non-interacting proteins (1° antibodies: VE–cadherin+actin; V+A) controls all showed negative signals. Quantification of red signals showed increased TiO2–NM interaction with VE–cadherin with increasing dose of TiO2–NM. Scale bar, 50 μm. Data are means±s.d. ofn=3. Student’st-test, compared with untreated control, *P<0.05. Figure 3: TiO 2 –NM directly bind to adherens junctional homophilic VE–cadherin. ( a ) The presence of TiO 2 –NM pulled down VE–cadherin (VEC) in a dose-dependent manner. Post lysis (P), addition of TiO 2 –NM (1,250 μM) to a non-treated control did not pull down any detectable VE–cadherin. This suggested that an intact adherens junction is important for TiO 2 –NM to bind to VE–cadherin. This showed that TiO 2 –NM binds to VE–cadherin within the adherens junction and not in the lysis buffer condition. Protein A Agarose beads (A) were added to show that no detectable VE–cadherin were precipitated without addition of TiO 2 –NM. Whole cell lysate showed similar expression of VE–cadherin across the various groups, which indicated that TiO 2 –NM did not affect cellular VE–cadherin expression transcriptionally or post-translationally. Schematic cartoon showing the experimental setup. ( b ) Direct interaction between TiO 2 –NM and VE–cadherin was assessed with modified PLA ( Supplementary Fig. S4 ). Intact monolayer of endothelial cells was treated with mouse-IgG-conjugated TiO 2 –NM for 30 min. Through the PLA protocol, red fluorescence signals were observed following mouse IgG-conjugated TiO 2 –NM treatments (100 and 250 μM), thus showing direct interaction. Untreated control, NM nonspecific control and non-interacting proteins (1° antibodies: VE–cadherin+actin; V+A) controls all showed negative signals. Quantification of red signals showed increased TiO 2 –NM interaction with VE–cadherin with increasing dose of TiO 2 –NM. Scale bar, 50 μm. Data are means±s.d. of n =3. Student’s t -test, compared with untreated control, * P <0.05. Full size image TiO 2 –NM trigger VE–cadherin pathway and actin remodelling TiO 2 –NM binding ( Fig. 3a , b) only partially explains the ECL phenomenon. Disruption alone does not account for gaps that were at least of micron separation distances as seen in the confocal images of leakiness ( Fig. 1a and Fig. 3b ). Activation of the VE–cadherin-mediated actin-rearrangement pathway explains the size of observed gaps. Based on the canonical VE–cadherin disruption pathway, an external ligand stimulus like VEGF or histamine activates phosphorylation of intracellular domain of VE–cadherin at its Y658 and Y731 residues [16] , [17] . Perimembraneous actin stability is linked to VE–cadherin’s intracellular domain through interactions with β-catenin and p120 [5] via these two phosphorylation sites. Cadherin–catenins–actin ternary complex has a pivotal role in cell shape and junction stability and endothelial permeability [5] . The phosphorylation at Y658 and Y731 signals the loss of VE–cadherin interaction with p120 and β-catenin, respectively, consequentially activating the actin remodelling pathway followed by the deformation of cell shape resulting in gaps between cells [5] . The manner which NM induced endothelial leakiness (NanoEL) appeared to be very different because it is unlikely that endothelial cells have evolved a cognate receptor for an artificial entity like a nanoparticle to bring about the NanoEL effect. Therefore, we asked to what degree of similarity does NM-induced endothelial leakiness coincide with the canonical ligand–receptor axis. We then showed that TiO 2 –NM treatment also resulted in phosphorylation outcomes reminiscent to that of VEGF and histamine ( Fig. 4a ). Guided by our VEGF- and histamine-mediated signalling data, we checked with a Src kinase inhibitor, PP1, whether Src kinase might be responsible for this TiO 2 -NM-induced phosphorylation ( Fig. 4a ). The inhibition of Src kinase with PP1 did not prevent the phosphorylation of the Y658 residue of VE–cadherin while the phosphorylation of the Y731 residue instead was repressed. As expected, inhibiting Src kinase with PP1 reduced the endothelial leakiness induced by VEGF and histamine [16] , [17] but did not have a significant effect on TiO 2 –NM-mediated leakiness ( Fig. 4a ). These observations suggested that a non-Src tyrosine kinase might be involved. Subsequently, immunoprecipitation results showed the loss of interaction between VE–cadherin with either β-catenin or p120 catenin as early as 15 min of TiO 2 –NM treatment ( Fig. 4b ). We next checked for internalization and degradation of VE–cadherin; events that are linked to the leakiness phenotype [18] . Consistent with observations from the treatment of VEGF and histamine, TiO 2 –NM stimulated the internalization of VE–cadherin ( Fig. 4c ) and its subsequent degradation ( Fig. 4c ). As observed earlier with the modified PLA technique, there were TiO 2 –NM interacting with VE–cadherin further inward from the cell surface ( Fig. 3b ). This suggested that TiO 2 –NM after binding with VE–cadherin might have followed VE–cadherin into the cytoplasm during the process of internalization of VE–cadherin. Taken together, we proposed that the disruption of homophillic interaction of VE–cadherin by TiO 2 –NM would trigger the machinery that leads to actin rearrangement resulting in changes to cell shape and therefore leakiness between neighbouring endothelial cells. To investigate whether perturbation of the cytoskeletal network can prevent TiO 2 –NM-induced leakiness, confluent layer of endothelial cells were pretreated with the RhoA kinase (ROCK) inhibitor, Y-27632 (5 and 10 μM), for 1 h. ROCK inhibits depolymerization of F-actin by myosin phosphotase and cofilin, resulting in the F-actin stabilization [19] . The inhibition of ROCK activity reduced the formation of stress fibres while maintaining the cell–cell adhesion, as shown by the VE–cadherin staining, without any apparent observable formation of intercellular gaps ( Fig. 4d ). In fact, transwell assay suggested that Y-27632 treatment actually enhanced endothelial barrier function by about twofold presumably via recruitment of F-actin to α- or β-catenin-containing junctions [20] . Interestingly, TiO 2 –NM treatment to Y-27632 preconditioned samples still led to an increase in dextran–FITC flux, albeit to a much lower level compared with the untreated Y-27632 control ( Fig. 4d ). These data showed that the perturbation of the cytoskeletal network was able to mitigate but unable to completely block TiO 2 –NM-induced ECL. This suggests that cytoskeletal remodelling is necessary and potentially a downstream event that facilitates the formation of TiO 2 –NM-induced micron-sized gaps. Overall, it was unexpected that TiO 2 –NM binding to VE–cadherin itself can trigger phosphorylation of VE–cadherin because a ligand–receptor mechanism was previously thought to be the trigger for the same phosphorylation outcomes. Our data further showed that the binding of a foreign entity, like a nanoparticle, can trigger the same outcome as VEGF or histamine, albeit through a yet unclear kinase-initiated cascade. This can still culminate to ECL. 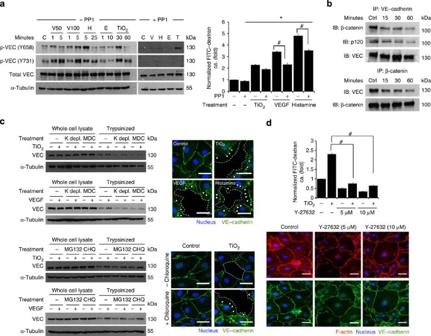Figure 4: TiO2–NM induce phosphorylation, internalization and degradation of VE–cadherin. (a) TiO2–NM treatment induced tyrosine phosphorylation of VE–cadherin at Y658 and Y731 but may not involve Src kinase. TiO2–NM (250 μM) triggered important Y658 and Y731 phosphorylation. VEGF (V), histamine (H) and EDTA (E) served as control stimulants. Src kinase inhibitor, PP1, effectively inhibited VEGF- and histamine-induced phosphorylation of VE–cadherin at Y658 and Y731. However, TiO2–NM treatment showed persistent phosphorylation of Y658 even with PP1 treatment. PP1 treatments were able to reduce the degree of FITC–dextran flux across the endothelial monolayer in VEGF- and histamine-treated samples. However in TiO2–NM case, dextran flux was relatively less repressed with PP1 treatment as compared with PP1 treatment in VEGF and histamine groups. Data are means±s.d. (n=3). Studentt-test,P<0.05 (*treated versus untreated control;#with PP1 versus without PP1). (b) TiO2–NM treatment induces release of p120 and β-catenin from VE–cadherin. Decreased interaction between VE–cadherin with β-catenin and between VE–cadherin with p120 following TiO2–NM treatment (250 μM). The vice versa immunoprecipitation of β-catenin also show decreased interaction with VE–cadherin. (c) TiO2–NM mediated internalization and degradation of VE–cadherin. Increased amount of internalized VE-cadherin was observed following TiO2–NM treatment. Potassium depletion (K depl.) and MDC further reduced internalization of VE–cadherin. Immunofluorescence helps to detect internalized VE–cadherin (white arrowheads) following treatment of TiO2–NM, VEGF or histamine, while for control group, VE–cadherin was confined to the cell boundaries. The cell periphery is demarcated by the dashed line. Scale bar, 15 μm. TiO2–NM treatment led to the lysosomal degradation of VE–cadherin. Inhibiting the proteasome pathway with MG132 did not result in any significant increase in the amount of VE–cadherin. In contrast, inhibiting the lysosomal pathway with chloroquine (CHQ) showed an increased stability of internalized VE–cadherin as shown in the western blot data and the confocal imaging of internalized VE–cadherin. (d) TiO2–NM activated actin remodelling that led to leakiness. ROCK inhibitor, Y-27632, treatment alone reduced inherent endogenous endothelial leakiness and negated TiO2-NM (250 μM)-induced leakiness. Treatment with Y-27632 for 1 h effectively abrogated formation of stress fibres without comprising endothelial barrier integrity as shown by the VE–cadherin staining. Scale bar, 20 μm. Data are means±s.d. (n=3). Student'st-test,P<0.05.#Significant difference against TiO2–NM treatment. Figure 4: TiO 2 –NM induce phosphorylation, internalization and degradation of VE–cadherin. ( a ) TiO 2 –NM treatment induced tyrosine phosphorylation of VE–cadherin at Y658 and Y731 but may not involve Src kinase. TiO 2 –NM (250 μM) triggered important Y658 and Y731 phosphorylation. VEGF (V), histamine (H) and EDTA (E) served as control stimulants. Src kinase inhibitor, PP1, effectively inhibited VEGF- and histamine-induced phosphorylation of VE–cadherin at Y658 and Y731. However, TiO 2 –NM treatment showed persistent phosphorylation of Y658 even with PP1 treatment. PP1 treatments were able to reduce the degree of FITC–dextran flux across the endothelial monolayer in VEGF- and histamine-treated samples. However in TiO 2 –NM case, dextran flux was relatively less repressed with PP1 treatment as compared with PP1 treatment in VEGF and histamine groups. Data are means±s.d. ( n =3). Student t -test, P <0.05 (*treated versus untreated control; # with PP1 versus without PP1). ( b ) TiO 2 –NM treatment induces release of p120 and β-catenin from VE–cadherin. Decreased interaction between VE–cadherin with β-catenin and between VE–cadherin with p120 following TiO 2 –NM treatment (250 μM). The vice versa immunoprecipitation of β-catenin also show decreased interaction with VE–cadherin. ( c ) TiO 2 –NM mediated internalization and degradation of VE–cadherin. Increased amount of internalized VE-cadherin was observed following TiO 2 –NM treatment. Potassium depletion (K depl.) and MDC further reduced internalization of VE–cadherin. Immunofluorescence helps to detect internalized VE–cadherin (white arrowheads) following treatment of TiO 2 –NM, VEGF or histamine, while for control group, VE–cadherin was confined to the cell boundaries. The cell periphery is demarcated by the dashed line. Scale bar, 15 μm. TiO 2 –NM treatment led to the lysosomal degradation of VE–cadherin. Inhibiting the proteasome pathway with MG132 did not result in any significant increase in the amount of VE–cadherin. In contrast, inhibiting the lysosomal pathway with chloroquine (CHQ) showed an increased stability of internalized VE–cadherin as shown in the western blot data and the confocal imaging of internalized VE–cadherin. ( d ) TiO 2 –NM activated actin remodelling that led to leakiness. ROCK inhibitor, Y-27632, treatment alone reduced inherent endogenous endothelial leakiness and negated TiO 2 -NM (250 μM)-induced leakiness. Treatment with Y-27632 for 1 h effectively abrogated formation of stress fibres without comprising endothelial barrier integrity as shown by the VE–cadherin staining. Scale bar, 20 μm. Data are means±s.d. ( n =3). Student's t -test, P <0.05. # Significant difference against TiO 2 –NM treatment. Full size image TiO 2 –NM cause ECL in subcutaneous blood vessels In vivo ECL can lead to edema owing to an increase in interstitial pressure. In extreme cases of ECL, cell–cell junctions are chronically disrupted resulting in extensive vascular damage. We chose two distinctly different mouse models to investigate whether TiO 2 –NM causes leakiness in an in vivo setting. To show that there is direct vascular leakiness, we injected either TiO 2 –NM or vehicle buffer into subcutaneous pockets created on the back of mice. The relatively sparse and distinct vascular network ( Fig. 5a ) reduced the chance of damaging the blood vessels solely due to injection [4] . We then injected Evan’s blue dye (EBD) into the tail vein and sacrificed the animals. We observed that TiO 2 –NM at a localized dose of 8 μg kg −1 mouse mass was sufficient to cause increased EBD extravasation at the subcutaneous vasculature on the back of mice ( Fig. 5b ). These results indicate that TiO 2 –NM can cause vascular leakiness in a localized delivery. 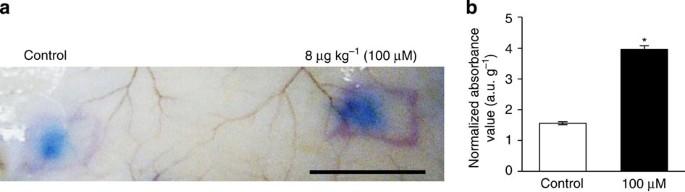Figure 5: TiO2–NM promote leakiness of subcutaneous blood vessel. (a) TiO2–NM were carefully injected into subcutaneous pockets on the back of mice. EBD was injected into circulation via tail-vein injection. (b) EBD extravasation was more pronounced in the TiO2–NM group (8 μg kg−1dose equivalent to 100 μM). Quantification of EBD showed more endothelial leakiness in the TiO2–NM group compared with the untreated mice group. Scale bar, 1 cm. Results represent for means±s.d. from three independent experiments, Student'st-test, *P<0.05 compared with untreated control. Figure 5: TiO 2 –NM promote leakiness of subcutaneous blood vessel. ( a ) TiO 2 –NM were carefully injected into subcutaneous pockets on the back of mice. EBD was injected into circulation via tail-vein injection. ( b ) EBD extravasation was more pronounced in the TiO 2 –NM group (8 μg kg −1 dose equivalent to 100 μM). Quantification of EBD showed more endothelial leakiness in the TiO 2 –NM group compared with the untreated mice group. Scale bar, 1 cm. Results represent for means±s.d. from three independent experiments, Student's t -test, * P <0.05 compared with untreated control. Full size image TiO 2 –NM cause ECL in a mouse lung metastasis model Pathological ECL can enhance tumour cell metastasis [4] . The tumour vasculature is often leaky, which increased nutrients flux to tumours. Leaky vasculature at secondary sites from the initial tumour sites, like distal organs, may act as exit points for metastatic circulating tumour cells, allowing secondary cancer colonization. Studies using inhalation and transdermal delivery of TiO 2 –NM resulted in accumulation in major organs like the liver, kidney and lungs [21] , [22] . We therefore reasoned that if accumulated TiO 2 –NM in lung tissue can cause aberrantly leaky blood vessels in the lung vasculature, we might observe higher metastasis of cancer cells. We used an established mouse model where B16F10 mouse melanoma cells injected into circulation metastasized to the lung and showed increased secondary metastatic colonization when there was increased vascular leakiness [4] , [23] , [24] , [25] . In an acute (1 week) high-dose TiO 2 –NM (50 and 150 mg TiO 2 –NM per kg mouse mass) exposure mouse model, we observed significantly more superficial melanoma-to-lung metastasis in the TiO 2 –NM-treated groups in a dose-dependent manner when compared with the control group ( Fig. 6 ). There were clear distinct colonies both on the surface and stroma of the lung lobes ( Fig. 6a ). The metastasis load within the lungs were quantified with quantitative PCR (qPCR) analysis for melanin A, a marker of melanoma cells ( Fig. 6c ), which showed increased melanoma metastasis to the lung in the TiO 2 –NM-treated groups. Scoring of histologically stained lung sections ( Fig. 6d ) showed significant increase of tumour penetration and tumour nodules formation with increasing dose of TiO 2 –NM ( Fig. 6d ). Percentage of lung section coverage by tumours was also significantly increased with increasing dose ( Fig. 6e ). 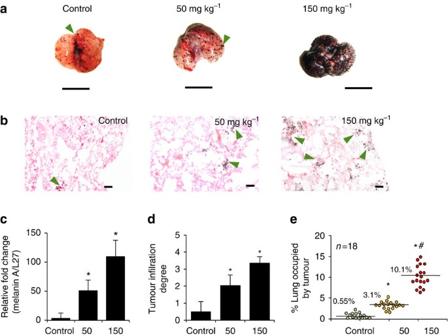Figure 6: TiO2–NM promote vessel leakiness in a melanoma-lung metastasis model. The mice were pre-injected with 106mouse melanoma cells (B16F10) and then with either TiO2–NM suspension 50 or 150 mg kg−1with repeat injections every other day and animals were sacrificed on the seventh day. (a) B16F10 in circulation were able to establish more colonies (green arrowheads) in lungs. There was a dramatic increase in superficial lung metastatic load from 50 to 150 mg TiO2–NM per kg mouse mass. Scale bar, 1 cm. (b) Eosin-stained sections of lungs showing melanoma colonies (green arrowheads). Scale bar, 50 μm. (c) qPCR analysis of lung tissues showed significant increase in melanin A expression with increasing dose of TiO2–NM treatment. Data shown were for means±s.d from triplicate qPCR reactions per individual lungs (n=3) in each group. Student’st-test, compared with untreated control *P<0.05. (d) Quantification of the degree of cancer metastasis through blinded scoring made by ten unbiased evaluators of six randomly selected sections per group (n=3 lungs per group). Data are means±s.d. Student’st-test, compared with untreated control *P<0.05. (e) Image analysis results quantifying percentage coverage of tumour area over lung section area (analysis steps inSupplementary Fig. S5)n=18 per group. Tumour area occupancy over lung section was found to significantly increase in a dose dependent manner upon TiO2–NM treatment. Student’st-test,P<0.05 (*treated versus untreated control, # 150 mg kg−1group versus 50 mg kg−1. Figure 6: TiO 2 –NM promote vessel leakiness in a melanoma-lung metastasis model. The mice were pre-injected with 10 6 mouse melanoma cells (B16F10) and then with either TiO 2 –NM suspension 50 or 150 mg kg −1 with repeat injections every other day and animals were sacrificed on the seventh day. ( a ) B16F10 in circulation were able to establish more colonies (green arrowheads) in lungs. There was a dramatic increase in superficial lung metastatic load from 50 to 150 mg TiO 2 –NM per kg mouse mass. Scale bar, 1 cm. ( b ) Eosin-stained sections of lungs showing melanoma colonies (green arrowheads). Scale bar, 50 μm. ( c ) qPCR analysis of lung tissues showed significant increase in melanin A expression with increasing dose of TiO 2 –NM treatment. Data shown were for means±s.d from triplicate qPCR reactions per individual lungs ( n =3) in each group. Student’s t -test, compared with untreated control * P <0.05. ( d ) Quantification of the degree of cancer metastasis through blinded scoring made by ten unbiased evaluators of six randomly selected sections per group ( n =3 lungs per group). Data are means±s.d. Student’s t -test, compared with untreated control * P <0.05. ( e ) Image analysis results quantifying percentage coverage of tumour area over lung section area (analysis steps in Supplementary Fig. S5 ) n =18 per group. Tumour area occupancy over lung section was found to significantly increase in a dose dependent manner upon TiO 2 –NM treatment. Student’s t -test, P <0.05 (*treated versus untreated control, # 150 mg kg −1 group versus 50 mg kg −1 . Full size image However, the TiO 2 –NM doses in this acute exposure study were very high and any longer experimentation lapsed into very low animal survival rates, making it difficult to study a more chronic treatment. To study subchronic treatment of TiO 2 –NM, we dropped the concentration by 30-fold to 5 mg kg −1 and injected a single bolus of 500,000 cells at the start of the third week and extended the TiO 2 –NM treatment to the end of 4 weeks. We included TiO 2 microparticles (680 nm) as another study group. Results showed the gross appearance of tumour nodules on the surface ( Fig. 7a ) and stroma of the lungs ( Fig. 7b ) from the TiO 2 –NM-treated group. qPCR analysis of melanin A in lung samples after TiO 2 –NM treatment showed an increased degree of metastatic colonization as compared with control and the microparticles groups ( Fig. 7c ). Histologically stained section scoring showed a similar trend of TiO 2 –NM increasing metastasis of melanoma cells ( Fig. 7d ) as compared with the control and microparticles groups. Percentage of lung section coverage by tumours was also significantly increased in the group with TiO 2 –NM treatment compared with the control and microparticles groups ( Fig. 7e ). 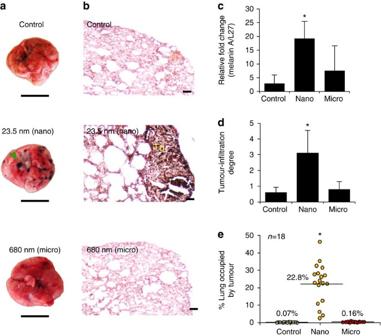Figure 7: Low-dose subchronic TiO2–NM treatment promote vessel leakiness. The mice were injected with either 5 mg/kg TiO2-NM, 10 mg/kg TiO2microparticles and vehicle control; total 7 boluses were given with each given every other day. 500,000 B16F10 melanoma cells injection was at 3rd week. Experiment was terminated at the end of 4 weeks. (a) Superficial images showing a dramatic increase in lung metastasis in the TiO2–NM group (23.5 nm) compared with control and microparticles (680 nm). Scale bar, 1 cm. (b) Eosin-stained sections of lungs of mice. Tumour nodule (Tu) indicated the presence of metastasized melanoma in the lung stroma. Scale bar, 50 μm. (c) qPCR analysis of melanoma tumours in lungs showed significant increase in melanin A expression with TiO2–NM treatment. Data are means±s.d. from three different lungs, *P<0.05 when compared with control, Student’st-test. (d) Assessments made by ten unbiased evaluators of six randomly selected sections per group (n=3 lungs per group). Data are means±s.d. Student’st-test, treated with NM compared with untreated control or treated with microparticles versus control, *P<0.05. (e) Image analysis results quantifying percentage coverage of tumour area over lung section area (analysis steps inSupplementary Fig. S5).n=18 per group. There was significantly higher area occupancy of tumours in the lung sections of the TiO2–NM-treated animals as compared with the control and TiO2microparticle-treated groups, Student'st-test,P<0.05 (*treated versus untreated control). Figure 7: Low-dose subchronic TiO 2 –NM treatment promote vessel leakiness. The mice were injected with either 5 mg/kg TiO 2 -NM, 10 mg/kg TiO 2 microparticles and vehicle control; total 7 boluses were given with each given every other day. 500,000 B16F10 melanoma cells injection was at 3rd week. Experiment was terminated at the end of 4 weeks. ( a ) Superficial images showing a dramatic increase in lung metastasis in the TiO 2 –NM group (23.5 nm) compared with control and microparticles (680 nm). Scale bar, 1 cm. ( b ) Eosin-stained sections of lungs of mice. Tumour nodule (Tu) indicated the presence of metastasized melanoma in the lung stroma. Scale bar, 50 μm. ( c ) qPCR analysis of melanoma tumours in lungs showed significant increase in melanin A expression with TiO 2 –NM treatment. Data are means±s.d. from three different lungs, * P <0.05 when compared with control, Student’s t -test. ( d ) Assessments made by ten unbiased evaluators of six randomly selected sections per group ( n =3 lungs per group). Data are means±s.d. Student’s t -test, treated with NM compared with untreated control or treated with microparticles versus control, * P <0.05. ( e ) Image analysis results quantifying percentage coverage of tumour area over lung section area (analysis steps in Supplementary Fig. S5 ). n =18 per group. There was significantly higher area occupancy of tumours in the lung sections of the TiO 2 –NM-treated animals as compared with the control and TiO 2 microparticle-treated groups, Student's t -test, P <0.05 (*treated versus untreated control). Full size image The tumours in the subchronic experiment were less numerous and larger ( Fig. 7b ) compared with the acute case ( Fig. 6b ) because the bolus of B16F10 metastatic melanoma cells are halved and were given twice as long to colonize and multiply. Overall, these mouse models again recapitulated the findings of the earlier described in vitro experiments that TiO 2 –NM increases ECL. In this report, we showed a novel non-receptor-mediated and direct binding mechanism of a dense and rigid NM entering into the adherens junction of endothelial cells and disrupting the interaction of VE–cadherin as the trigger for ECL. This is in stark contrast to the better understood receptor-mediated mechanism of inducing ECL through binding of a mediator molecule to its receptor with examples like thrombin with PAR-1; bradykinin with bradykinin receptors β1, 2 and 3; histamine with H1 receptors; VEGF and its receptors, VEGFR-1 and VEGFR-2 [26] . Chemical-mediated mechanisms that can trigger ECL include oxidative stress and endotoxin though both these cases require cellular uptake of substances [27] , [28] and ECL is a secondary effect. It is still unknown how the adherens junction is targeted by a nanoparticle in the first place though we postulate that the negatively charged glycocalyx found on the luminal side of endothelial cells may have repelled the sedimenting negatively charged corona-coated TiO 2 –NM ( Supplementary Fig. S1 ) and coupled together with a high mass density; TiO 2 –NM might have ‘bounced and rolled’ into the adherens junction and entrapped within the confines of the adherens junction niche. The current paradigm of how NM cross cell barriers is through a series of steps; (a) crossing the cell membrane, (b) endocytosis, (c) intracellular trafficking, (d) repackaging into exocytotic vesicles and (e) traversing the cell membrane [28] . What we have found is novel and in stark contrast to this prevailing paradigm. The traversing of the mono endothelial cell layer via the route through the adherens junction logically presents less impedence to the nanoparticle. After leakiness is established, this route between the adherens junction allows the ‘nano-exodus’ of more NM across the endothelium. Therefore, we coined this effect as ‘nanomaterials induced endothelial leakiness’ (NanoEL). Exactly how this disruptive binding of TiO 2 –NM to VE–cadherin occurs is unknown. As we have shown that negatively charged TiO 2 –NM ( Supplementary Fig. S1 ) binds directly to VE–cadherin, it can either bind directly to the extracellular domains where homophilic interaction occurs [29] and disrupts that interaction, or the other domains of VE–cadherin not involved in the homophilic interaction or even the Ca 2+ ions itself. EDTA disrupts homophilically interacting VE–cadherin by chelating Ca 2+ ions [4] . That may provide clues that negatively charged TiO 2 –NM with protein corona ( Supplementary Fig. S1 ) may have bound to positively charged side chains of VE–cadherin that rigidity of VE–cadherin is compromised [30] . The loss in rigidity in VE–cadherin or even denaturation of VE–cadherin [31] may have caused the loss in homophilic interaction. Whichever the case is, mechanical perturbation at the VE–cadherin molecular scale may actually induce the cascade that leads to leakiness. This notion is supported by a study showing that macroscopic hydrodynamic stress on endothelial cells could bring about phosphorylation of VE–cadherin [32] . We further reinforce the idea that mechanical perturbation may drive a different kinase pathway from ligand–receptor-based induction but still converges to the canonical axis of phosphorylation of VE–cadherin. Our observations have opened up the exciting possibility of VE–cadherin molecule itself as a direct stress sensor. We only showed that three NM (primary size range 15–25 nm) causes ECL, and more investigation needs to be carried out in determining whether this effect is also observed in other similarly sized nanoparticles of other materials. If the ECL-inducing phenomenon is more universal than what we have showed with three different NM, it is then important to also check whether nanomedicine itself causes ECL. Nanomedicine as anticancer drugs act at the molecular level with promising applications in clinics [33] . While tumours have leaky blood vessels that have enhanced permeability and retention effects (EPR), circulating nanomedicine intentionally introduced into the vascular system may also inevitably accumulate unintentionally in other non-tumour sites of major organs. While EPR effect can explain metastasis at the primary site of the tumour, based on our study, NM accumulation at non-tumour sites may lead to enhanced secondary metastasis to those sites through NanoEL effects. We have shown in this study that TiO 2 –NM may have detrimental effects; however, the same properties can also be capitalized in nanomedicine, used in situations where leakiness is therapeutic. Situations like traversing the blood–brain barrier by inducing vascular leakiness to facilitate a lower dose of drugs to the brain though the nonspecific accumulation issue still needs to be resolved. Overall, determination of this size–charge–mass density window will equip nano-biotechnologists with rules to engineer NM that either avoid or capitalize on this NanoEL effect. Our mode of TiO 2 –NM delivery in the mouse experiments is artificial because the situations where TiO 2 –NM is intentionally introduced directly into the bloodstream would be very rare. While we want to emphasize that these mouse studies are ‘proof of concept’ experiments and not indicative of real human situations, we would also argue for the need of such controlled animal experiments so we can understand the risk of NM. There are no published reports on TiO 2 –NM-controlled human exposures without any confounding factors over a long period of time and quantification of TiO 2 –NM accumulation in all the major organs. Mouse studies, however, involving respiratory and dermal introduction of TiO 2 –NM did show a low percentage (lung accumulation estimate of 0.003%) of traversing the various barriers to reach and accumulate in the major organs [21] , [22] . Occupational inhalation of manufactured TiO 2 –NM and its corresponding accumulation in the lungs is high with a comparatively low clearance rate [34] . Deducing from these studies, one can surmise that if given enough exposure time, dose and frequency, it is possible to reach doses that may cause NanoEL. In addition, the pre-existing diseased conditions that increase vascular permeability, like infection [35] , may exacerbate the onset of NanoEL effect. We, however, need to point out that in order to reach those doses used in our study, we would require extreme circumstances of long-term chronic exposures across possibly damaged epithelia [36] . In conclusion, we have described a novel observation that TiO 2 –NM causes ECL and showed that the mechanism preceded oxidative stress. Our data suggest and support a novel mechanism that TiO 2 –NM being small enough to migrate into the inter-endothelial adherens junction niche, binds directly to VE–cadherin and disrupts these cell–cell interactions. This disruption leads to the phosphorylation of intracellular VE–cadherin, which in turn resulted in loss of interaction between intracellular domains of VE–cadherin with β-catenin and with p120, triggering the unintended avalanche of actin-rearrangement pathway, which eventually brought about ECL (mechanism summarized in Fig. 8 ). The fate of VE–cadherin appears to follow the canonical ligand–receptor-mediated pathway where VE–cadherin may be internalized and degraded. We have also demonstrated that TiO 2 –NM may cause NanoEL effects resulting in enhanced circulating melanoma metastasis to the lungs. In addition, this study emphasizes the importance of understanding NM interactions with biological systems and especially extracellular niches. 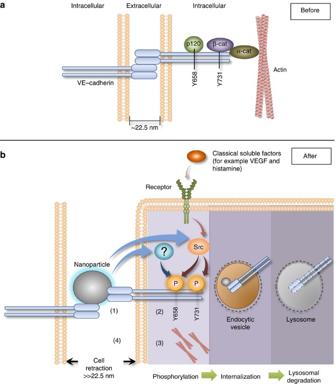Figure 8: Proposed mechanism of TiO2NanoEL. (a) The anatomy of an adherens junction. Intact monolayer of connected endothelial cells is maintained by stable VE–cadherin homophilic interactions with neighbouring cells. VE–cadherin forms atrans-homophillic interaction at the EC domains with anothercis-paired VE–cadherin complex. β-catenin, p120 and VE–cadherin form a complex. Formation of this ternary complex stabilizes the adherens junction38. Distance of adherens junction is at least 22.5 nm. (b) TiO2–NM are small enough to migrate into the adherens junction; they bind and disrupt VE–cadherin homophilic interaction (1). This disruption induces the phosphorylation of Y658 of VE-cadherin via a currently unknown kinase pathway, while the Y731 residue is phosphorylated by Src kinase. The phosphorylation at the two residues induces the loss of interaction between VE–cadherin and β-catenin and with p120 (2). The loss of interaction of the VE–cadherin–β-catenin–p120 complex destabilizes actin and lead to actin remodelling (3). As a result the cell retracts and leakiness occurs (4). After the binding of TiO2-NM to VE–cadherin, VE–cadherin might be internalized and further degraded by lysosomes. Fate of VE–cadherin: phosphorylation of VE–cadherin due to NanoEL may result in internalization and lysosomal degradation. This minimizes the overall amounts of VE–cadherin near the vicinity of the cell membrane. TiO2–NM might be internalized alongside VE–cadherin as it remained bound to VE–cadherin but the final fate of the TiO2–NM is uncertain. Figure 8: Proposed mechanism of TiO 2 NanoEL. ( a ) The anatomy of an adherens junction. Intact monolayer of connected endothelial cells is maintained by stable VE–cadherin homophilic interactions with neighbouring cells. VE–cadherin forms a trans -homophillic interaction at the EC domains with another cis -paired VE–cadherin complex. β-catenin, p120 and VE–cadherin form a complex. Formation of this ternary complex stabilizes the adherens junction [38] . Distance of adherens junction is at least 22.5 nm. ( b ) TiO 2 –NM are small enough to migrate into the adherens junction; they bind and disrupt VE–cadherin homophilic interaction (1). This disruption induces the phosphorylation of Y658 of VE-cadherin via a currently unknown kinase pathway, while the Y731 residue is phosphorylated by Src kinase. The phosphorylation at the two residues induces the loss of interaction between VE–cadherin and β-catenin and with p120 (2). The loss of interaction of the VE–cadherin–β-catenin–p120 complex destabilizes actin and lead to actin remodelling (3). As a result the cell retracts and leakiness occurs (4). After the binding of TiO 2 -NM to VE–cadherin, VE–cadherin might be internalized and further degraded by lysosomes. Fate of VE–cadherin: phosphorylation of VE–cadherin due to NanoEL may result in internalization and lysosomal degradation. This minimizes the overall amounts of VE–cadherin near the vicinity of the cell membrane. TiO 2 –NM might be internalized alongside VE–cadherin as it remained bound to VE–cadherin but the final fate of the TiO 2 –NM is uncertain. Full size image Functionalization of TiO 2 –NM FITC was covalently tagged to TiO 2 –NM P25 (Evonik Degussa, USA). Briefly, 100 mg of TiO 2 –NM were dispersed in 100 ml of anhydrous ethanol (Fisher Scientific, USA); thereafter 5 ml of aminopropyltriethoxysilane (APTES, Sigma Aldrich, USA) was added to the suspension and stirred at 80 °C for 3 h. Then, 25 mg of FITC was added to the mixture and was stirred for another 16 h at 80 °C. The FITC-tagged TiO 2 was collected, and thoroughly washed with ethanol and subsequently with ultrapure water. To conjugate mouse IgG to TiO 2 –NM, 10 mg of silanized TiO 2 –NM (after treatment with APTES) was activated with 1.5 ml of 8% glutaraldehyde (Sigma Aldrich) for 6 h in room temperature. Thereafter, the activated TiO 2 –NM were collected, washed thrice with PBS and resuspended in 4 ml of PBS. One hundred and sixty microlitre of suspension (consisting of 400 μg of activated TiO 2 –NM) were added to 1 ml of PBS solution mouse IgG (20 μg; Millipore, USA). The mixture then was gently agitated for 16 h in 4 °C. Following the conjugation process, the mouse IgG-conjugated TiO 2 –NM were collected and washed thrice with PBS. The mouse IgG-conjugated TiO 2 –NM were resuspended in PBS solution and stored in 4 °C until further use. Proximity ligation assay PLA semiquantification was done by introducing mouse IgG-conjugated TiO 2 –NM to a monolayer HMVEC culture. Conjugation scheme is found in Supplementary Fig. S4 . Following treatment, the cells were washed thrice with PBS and fixed with 4% paraformaldehyde. Cell cytoplasm were visualized with Alexa 488 Actin staining (1:40; Invitrogen, USA) and the detection of PLA signal was done as per supplier instructions (Olink Bioscience, Sweden). The PLA signals were quantified with Duolink ImageTool software (Olink Bioscience) and normalized against the cell number ( n =25). Permeability transwell assay The degree of ECL was measured in Transwell insert (with polycarbonate filter, 0.4 μm pore; Corning Costar, Cambridge, MA) as described earlier [37] . Briefly, HMVEC were cultured with density of 20,000 cells per well for 2 days to achieve a confluent monolayer. Thereafter, FITC-dextran (1 mg ml −1 , average MW=40,000; Sigma Aldrich, USA) along with NM or microparticles suspension were added to cells.. At the end of treatment time (30 min), 100 μl samples were taken from the lower compartment and the fluorescence signal was quantified with a microplate reader at excitation/emission wavelength of 492/520 nm. Treatment of 2.5 mM EDTA was introduced as positive control. Immunofluorescence staining Cell junctions were visualized by immunofluorescence staining of VE–cadherin (Cell Signaling Technology, USA). HMVEC were grown overnight on 8-well chamber slides at initial seeding density of 4 × 10 4 cells per cm 2 . The cells were treated by replacing the growth medium with medium containing TiO 2 –NM. Following the treatment at various time points, media were removed and cells were gently washed with PBS. Thereafter, cells were fixed with 4% paraformaldehyde for 15 min, permeabilized using 0.2% Triton X-100 for 15 min and blocked for 1 h with 2% bovine serum albumin (BSA), 0.1% Triton X-100 in PBS. Fixed cells were incubated overnight at 4 °C with anti VE-cadherin antibody (1:200; Cell Signaling Technology) in 0.2% BSA. Thereafter, the cells were washed thrice with PBS, and incubated for 1 h at room temperature with Alexa 488-chicken anti rabbit antibody (1:400; Invitrogen). Finally, the labelled slides were mounted using ProLong Gold antifade reagent with 4',6-diamidino-2-phenylindole (Invitrogen). Images were obtained using Nikon A1 confocal microscope (Nikon, Japan). VE–cadherin internalization assay was performed in accordance to previous report [39] . Briefly, confluent HMVECs were serum starved for 6 h. At 3 h into the serum starvation, chloroquine (150 μM) was added to prevent lysosomal degradation of the internalized VE–cadherin. Cells were subsequently incubated with VE–cadherin BV6 (1:100; Millipore, 50 μg ml −1 ) antibody in medium containing 3% fetal bovine serum at 4 °C for 1 h. VE–cadherin BV6 antibody specifically recognizes the extracellular domain of VE–cadherin. Cells were then rinsed with ice-cold serum-free medium to remove excess unbound antibodies and then treated with the various stimuli for 30 min at 37 °C. Cells were washed with mild acidic buffer (pH 2.7) containing 3% BSA and 25 mm glycine in order to remove surface-bound VE–cadherin. Thereafter, the cells were washed and processed for immunofluorescence staining. TiO 2 –NM internalization study HMVEC were grown overnight either on 8-well chamber slides or 24-well plates at a seeding concentration of 4 × 10 4 cells per cm 2 . The inhibition of TiO 2 –NM endocytosis was done by pretreating the monolayer endothelial cells for 1 h with either 10 μM of monodansylcadaverine (MDC; Sigma Aldrich) or 5 mM methyl-β-cyclodextrin (MβCD; Sigma Aldrich) before TiO 2 –NM treatment. In order to measure the TiO 2 –NM uptake after endocytosis pathway is blocked, the cells were treated with FITC-TiO 2 NM (50 and 250 μM) for different time periods (30, 60 and 120 min). Subsequently, the cells were washed and lysed and the FITC signal was measured as mentioned before. In order to study the leakiness after endocytosis pathway is blocked, the monolayer HMVEC is treated with TiO 2 NM (50 and 250 μM) for 30 min. Later, the cells were washed and fixed with 4% paraformaldehyde before immunostaining as mentioned above. Separation of membrane-bound and cytosolic FITC–TiO 2 HMVEC were grown overnight on 6-cm culture dishes. FITC–TiO 2 –NM in EndoGRO complete medium were introduced to the cells and media was removed after various time points. For the control plate, FITC–TiO 2 –NM were added to the cells and immediately removed. After removal of media, cells were immediately washed thrice with PBS and detached from the culture dish. 10 6 cells were collected for further processing. Membrane and cytosolic fractions were separated by Mem-PER Eukaryotic Membrane Protein Extraction Kit (Thermo Scientific, USA). The FITC signals in the separated fractions were measured at excitation/emission wavelengths of 488/520 nm using Tecan Infinite 200 microplate reader (Tecan Inc., Switzerland). ROCK inhibition assay HMVEC seeded at an initial seeding density of 4 × 10 4 cells per cm 2 either in 8-well chamber slides or 24-well transwells and grown till confluent in EndoGRO complete medium. Confluent HMVEC were then rinsed three times with PBS and serum starved for 6 h at 37 °C, 5% CO 2 , following which cells were pretreated with Y-27632 ROCK inhibitor (5 and 10 μM) for 1 h before the addition of TiO 2 –NM. At 30 min post TiO 2 –NM treatment, cells were either processed for immunostaining or subjected to transwell assay. In vivo subcutaneous vascular leakiness assay Experimental protocols were approved by Nanyang Technological University Institutional Animal Care and Use Committee (A-0174AZ). Three-weeks-old BALB/c white mice were anesthetized and injected with either TiO 2 –NM or vehicule buffer (3% BSA in PBS). In order to determine the vascular permeability, Evans blue dye (Sigma-Aldrich, USA) was injected into the tail vein. Injection sites were randomly chosen to avoid biasness. The mice were sacrificed after 15 min and thereafter the skin was excised and the extravasated dye was extracted. Finally, the amount was quantified by measuring absorbance at 624 nm with microplate reader (Tecan Inc.). The absorbance measured was normalized to the weight of the skin excised. In vivo murine melanoma-lung metastasis model For acute study, wild-type C57BL/6J mice were intravenously injected with 10 6 cells melanoma (B16F10) cells (ATCC: CRL-6475). The mice were treated either with vehicle control in 1% BSA in PBS or with TiO 2 -NM suspended in 1% BSA in PBS (50, 150 mg kg −1 ). NM samples were freshly prepared and were intravenously injected into each mouse every 2 days from Day 0. Mice were sacrificed and the lungs were collected for further analysis. For subchronic study, wild-type C57BL/6J mice were divided into three groups of treatment. One group received 1% BSA in PBS (vehicle control), another received 5 mg kg −1 TiO 2 -NM and the last group received 10 mg kg −1 of TiO 2 microparticles. All TiO 2 materials were freshly prepared before intravenous injection. Five hundred thousand murine melanoma cells were intravenously injected. Total cellular RNA was extracted from the lung samples using the RNeasy fibrous tissue mini kit (Qiagen, USA) according to the recommended protocol. The extracted RNA was reverse transcribed to complementary DNA using RevertAid H-Minus First Strand cDNA Synthesis kit (Fermentas, USA), and the metastasis burden was quantified with qPCR of melanin A. The qPCR reactions were performed on ABI 7300 Prism system (Applied Biosystem, USA) using the SYBR Fast Universal qPCR kit (KAPA Biosystems, USA). Lung samples were fixed with 4% paraformaldehyde and stored at −80 °C with O.C.T. Tissue Freezing Compound (Leica Microsystems, USA). Fixed lung samples were cryosectioned at a thickness of 10 μm (Leica Microsystems CM1850, USA). The sections were stained with eosin (Sigma-Aldrich). The sections were then blind-scored by ten independent assessors. The degree of melanoma infiltration was scored with 5 and 0 as the highest and lowest, respectively. Statistical analysis Statistical significance was ascertained through Student’s t -test with SPSS software (SPPS16.0). P -value of <0.05 is considered significant. How to cite this article: Setyawati M.I. et al . Titanium dioxide nanomaterials cause endothelial cell leakiness by disrupting the homophilic interaction of VE-cadherin. Nat. Commun. 4:1673 doi: 10.1038/ncomms2655 (2013).